Critical roles for EphB and ephrin-B bidirectional signalling in retinocollicular mapping Graded expression of EphB and ephrin-B along the dorsoventral axis of the retina indicates a role for these bidirectional signalling molecules in dorsoventral–mediolateral retinocollicular mapping. Although previous studies have implicated EphB2 forward signalling in mice, the intracellular component of EphB2 essential for retinocollicular mapping is unknown as are the roles for EphB1, ephrin-B1, and ephrin-B2. Here we show that EphB2 tyrosine kinase catalytic activity and EphB1 intracellular signalling are key mediators of ventral–temporal retinal ganglion cell axon retinocollicular mapping, by likely interacting with ephrin-B1 in the superior colliculus. We further elucidate roles for the ephrin-B2 intracellular domain in retinocollicular mapping and present the unexpected finding that both dorsal and ventral–temporal retinal ganglion cell axons utilize reverse signalling for topographic mapping. These data demonstrate that both forward and reverse signalling initiated by EphB:ephrin-B interactions have a major role in dorsoventral retinal ganglion cell axon termination along the mediolateral axis of the superior colliculus. Retinal ganglion cells (RGCs), distributed along the dorsoventral axis of the retina, extend axons that terminate along the mediolateral axis of the superior colliculus (SC), whereas those distributed along the nasotemporal axis of the retina terminate along the rostrocaudal axis [1] , [2] . As they project along the SC rostrocaudal axis, RGC axons extend interstitial branches along the mediolateral axis that orient themselves towards their future termination zone (TZ) utilizing both repulsive and attractive mechanisms [2] . Ryk:Wnt3 signalling likely mediates the repulsion underlying mediolateral interstitial branch direction [3] , whereas the B-subclass Eph/ephrin molecules are thought to serve as an attractive counterbalance to these signals [4] . Ventral–temporal (VT) RGC axons of EphB2 −/− ;EphB3 −/− and EphB2 lacZ/lacZ ;EphB3 −/− compound mutants exhibited misprojecting interstitial branches that formed lateral biased ectopic TZs (eTZs) in the SC demonstrating a role for EphB:ephrin-B forward signalling in retinocollicular mapping. However, many questions remain about the individual contribution of EphB2 and EphB3 and a potential role for the related EphB1 receptor. Despite its robust VT retinal expression and key role in mediating axonal repulsion at the optic chiasm to form the ipsilateral projections essential for binocular vision [5] , nothing is known regarding how EphB1 participates in retinocollicular mapping. Likewise, despite the high dorsal/low ventral gradient of ephrin-B2 in the retina and elevated midline expression of ephrin-B1 in the SC [4] , the functions of these two molecules in mice are unknown. Using a diverse array of targeted mutations, we report here that EphB1 and EphB2 are the chief guidance molecules that mediate VT RGC axon targeting to the medial-rostral SC and that EphB2 tyrosine kinase catalytic activity is necessary. Genetic studies further demonstrated that ephrin-B1 is the primary ligand expressed in the SC for the mapping of VT RGC axons expressing EphB receptors. Finally, we show that reverse signalling mediated by high dorsal/low ventral expressed ephrin-B2 is important for retinocollicular mapping throughout the dorsoventral axis of the retina. Our study thus establishes the essential roles for both EphB1/EphB2 forward signalling and ephrin-B2 reverse signalling in guiding RGC axons to their proper TZ in the SC. EphB and ephrin-B expression in the retina and SC EphB2 expression in coronal sections of the retina and SC was confirmed using X-gal stains of EphB2 lacZ mutants, which express a carboxy-terminal truncated EphB2–β-gal fusion protein lacking the majority of the EphB2 intracellular domain including its tyrosine kinase catalytic domain, sterile alpha motif domain, and PSD95/Dlg/ZO1 (PDZ) binding motif [6] . This protein correctly traffics to the cell membrane and can act like a ligand to bind ephrin-B on adjacent cell surfaces to activate reverse signalling, but cannot transduce canonical forward signals into its own cell requiring the removed internal sequences. EphB2–β-gal expression visualized using X-gal staining matches both EphB2 expression visualized using anti-EphB2 antibody and EphB2 messenger RNA expression, as shown in embryonic and postnatal retinas, respectively [4] , [6] . The EphB2–β-gal fusion protein illustrates endogenous EphB2 protein expression in a high ventral/low dorsal gradient in the RGC layer at embryonic day 17.5 (E17.5) and postnatal days 1 (P1) and 8 (P8), although there is obvious expression in the dorsal retina ( Fig. 1a ). The localization of EphB2–β-gal at these stages is highly enriched in the RGC axons funneling into the optic nerve head (arrowheads in Fig. 1a ), as previously documented with EphB2 antibodies to detect the endogenous wild type (WT) protein [6] . In the brain, expression of EphB2 is also strong in the superficial and deeper layers of the SC at P1 and P8, but not in any visible gradient ( Fig. 1a ). 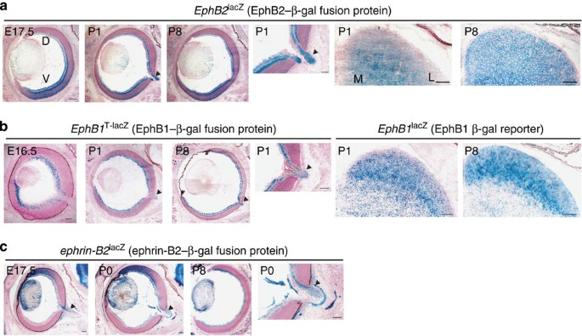Figure 1: EphB and ephrin-B expression in the retina and SC. (a)EphB2lacZmutants express a C-terminal, intracellular truncated EphB2–β-gal fusion protein that reaches the cell membrane and traffics to its normal cellular locations. X-gal stains of coronal sections from an E17.5 embryo, and P1 and P8 pups show EphB2 is expressed in a high ventral/low dorsal gradient in the retina and is localized to RGC axons that funnel into the optic nerve (arrowheads). EphB2–β-gal fusion protein is expressed uniformly in the SC at P1 and P8. (b)EphB1T-lacZmutants express a C-terminal, intracellular truncated EphB1–β-gal fusion protein that reaches the cell membrane and traffics to its normal cellular locations. X-gal stains of coronal sections from an E16.5 embryo, and P1 and P8 pups show EphB1 is highly expressed in the VT region of the embryonic retina, becoming more uniformly distributed at postnatal stages, and is localized to RGC axons that funnel into the optic nerve (arrowheads).EphB1lacZmutants express unconjugated β-gal in the cell body, and X-gal stains here show strong uniform expression within cells of the SC. (c)Ephrin-B2lacZmutants express a C-terminal, intracellular truncated ephrin-B2–β-gal fusion protein that reaches the cell membrane and traffics to its normal cellular locations. X-gal stains of coronal sections from an E17.5 embryo, and P0 and P8 pups show ephrin-B2 is expressed in a high dorsal/low ventral gradient in the retina and is localized to RGC axons that funnel into the optic nerve (arrowheads). Scale bar, 100 μm. D, dorsal; V, ventral; M, medial; L, Lateral. Figure 1: EphB and ephrin-B expression in the retina and SC. ( a ) EphB2 lacZ mutants express a C-terminal, intracellular truncated EphB2–β-gal fusion protein that reaches the cell membrane and traffics to its normal cellular locations. X-gal stains of coronal sections from an E17.5 embryo, and P1 and P8 pups show EphB2 is expressed in a high ventral/low dorsal gradient in the retina and is localized to RGC axons that funnel into the optic nerve (arrowheads). EphB2–β-gal fusion protein is expressed uniformly in the SC at P1 and P8. ( b ) EphB1 T-lacZ mutants express a C-terminal, intracellular truncated EphB1–β-gal fusion protein that reaches the cell membrane and traffics to its normal cellular locations. X-gal stains of coronal sections from an E16.5 embryo, and P1 and P8 pups show EphB1 is highly expressed in the VT region of the embryonic retina, becoming more uniformly distributed at postnatal stages, and is localized to RGC axons that funnel into the optic nerve (arrowheads). EphB1 lacZ mutants express unconjugated β-gal in the cell body, and X-gal stains here show strong uniform expression within cells of the SC. ( c ) Ephrin-B2 lacZ mutants express a C-terminal, intracellular truncated ephrin-B2–β-gal fusion protein that reaches the cell membrane and traffics to its normal cellular locations. X-gal stains of coronal sections from an E17.5 embryo, and P0 and P8 pups show ephrin-B2 is expressed in a high dorsal/low ventral gradient in the retina and is localized to RGC axons that funnel into the optic nerve (arrowheads). Scale bar, 100 μm. D, dorsal; V, ventral; M, medial; L, Lateral. Full size image To determine EphB1 expression in the retina and SC, two different EphB1 knock-in reporter lines expressing β-gal were used. In EphB1 lacZ mutants [5] , homologous recombination was used to insert a sa-IRES-lacZ cassette into EphB1 reading frame at exon 3 resulting in a protein-null mutation that also expresses a cytoplasmic β-gal reporter in cells that normally express EphB1 . In EphB1 T-lacZ mutants [7] , lacZ sequences were inserted in-frame into exon 9, directly after the transmembrane sequences, truncating the entire intracellular domain of the protein to express an EphB1–β-gal fusion protein. Similar to the EphB2–β-gal fusion protein, the EphB1–β-gal fusion also traffics normally to the cell membrane. X-gal stains for the EphB1 T-lacZ mutant reporter faithfully documented robust VT expression of EphB1 in the RGC layer at E16.5 whereas the dorsal and ventral-nasal retina expressed EphB1 at lower levels ( Fig. 1b ). EphB1 mRNA expression data at various embryonic stages also validates the X-gal patterns observed here [5] . By the first postnatal week, EphB1 expression loses its gradient and becomes expressed uniformly as shown at P1 and P8 using the EphB1 T-lacZ allele ( Fig. 1b ). EphB1–β-gal fusion protein was expressed in the RGC axons exiting into the optic nerve (arrowheads in Fig. 1b ). The EphB1 lacZ mutant reporter was used to assess EphB1 expression in the SC as the expression of unconjugated β-gal labels primarily cell bodies of expressing cells and not their processes. Here again, like EphB2, strong EphB1 expression was detected in the cells of the superficial and deeper layers of the SC at P1 and P8, and did not form a detectable gradient ( Fig. 1b ). Ephrin-B2 expression was determined using ephrin-B2 lacZ mutant mice, which express a C-terminal truncated ephrin-B2–β-gal fusion protein that lacks the intracellular segment [8] . The ephrin-B2–β-gal fusion protein is able to traffic to the cell membrane and bind Eph receptors on adjacent cells to activate forward signalling, but it is unable to transduce reverse signals into its own cell. X-gal stains of ephrin-B2 lacZ mice revealed a robust high dorsal/low ventral gradient expression of ephrin-B2–β-gal fusion protein in the RGC layer at E17.5, P0, and P8 ( Fig. 1c ), which complements previous mRNA expression data [4] , [9] . While the ephrin-B2–β-gal fusion protein was observed to be most intense in the dorsal retina, ventral expression was also evident at E17.5 and this became more obvious during the first postnatal week as seen at P0 and P8. The ephrin-B2–β-gal fusion protein is also particularly evident in axons leaving the dorsal retina as they form the optic nerve (arrowheads in Fig. 1c ). EphB2 forward signalling alone is needed for VT axon mapping Hindges et al . [4] previously reported significant retinocollicular mapping errors in EphB2 −/− ;EphB3 −/− and EphB2 lacZ/lacZ ;EphB3 −/− compound mutants, but did not analyse EphB2 single mutants to determine the contribution of this receptor separately from EphB3. Therefore, DiI was focally injected into the dorsal or VT retina to anterograde label RGCs so that formation of their TZs could be analysed at P8 ( Fig. 2a ). Also shown is an example of how a focal injection into the dorsal retina labels a TZ in the lateral SC of a WT mouse. Likewise, a focal injection into the VT retina illustrates the typical TZ size and medial-rostral location in a WT mouse, accompanied by the retinal flatmount to document the injection site ( Fig. 2b ). Of a total of 109 WT mice injected in the VT retina in our study, only 3 (<3%) formed an eTZ and of a total of 87 WT mice injected into the dorsal retina, only 1 (1%) of the SC formed an eTZ. In our analysis, the SC for each specimen that formed one or more eTZ had its primary and secondary TZs outlined, and then these images were superimposed according to genotype with the primary TZ positioned at the crosshairs of the compass as observed for the three WT ventral injected retinas that showed termination errors ( Fig. 2b ). The schematic summary allows for the qualitative assessment of the localization of the eTZs relative to the primary TZ. 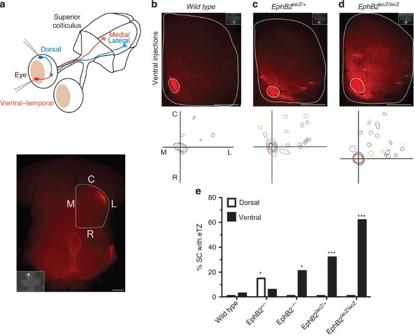Figure 2: EphB2 forward signalling alone is important for topographic mapping of RGC axons from the VT retina. (a) Top, schematic of the site of DiI injection in the dorsal or VT eye labelling RGCs and the expected TZ for their axonal projections in the lateral or medial contralateral SC, respectively. Bottom, dorsal view of a midbrain whole-mount depicting a normal TZ in the lateral SC from a WT mouse injected with DiI in the dorsal retina as verified in the flatmount (insert) and viewed using epifluorescence microscopy. (b) Top, example of a retina flatmount (insert) and SC whole mount from a WT mouse injected with DiI in the VT retina. Of 109 injected WT specimens analysed, only 3 formed one or more eTZs (3%). Bottom, the SC for each specimen that formed at least one eTZ had their eTZs and corresponding primary TZ outlined in the same colour. All outlines of the same genotype, in this case WT, were then superimposed on each other with the primary TZ positioned at the crosshairs of the compass as illustrated. (c) VT injectedEphB2lacZ/+heterozygotes formed eTZs (arrows) in 7/22 SC analysed. (d) VT injectedEphB2lacZ/lacZhomozygotes formed eTZs (arrows) in 8/13 SC analysed. (e) Graphic summary of the percent of SC that formed eTZs in mice injected with DiI in the dorsal or VT retina. Dorsal injected: WT (1%,n=87),EphB2+/−(15%,P=0.0437,n=13),EphB2−/−(0%,n=3),EphB2lacZ/+(0%,n=35), andEphB2lacZ/lacZ(0%,n=25). VT injected: WT (3%,n=109),EphB2+/−(6%,n=16),EphB2−/−(21%,P=0.0194,n=14),EphB2lacZ/+(32%,P=0.0001,n=22), andEphB2lacZ/lacZ(62%,P<0.0001,n=13). FET compared mutant groups with WT mice. Statistical significance is denoted by asterisks: *P≤0.05; **P≤0.01, and ***P≤0.001. Scale bar, 500 μm. C, caudal; L, lateral; M, medial; R, rostral. Figure 2: EphB2 forward signalling alone is important for topographic mapping of RGC axons from the VT retina. ( a ) Top, schematic of the site of DiI injection in the dorsal or VT eye labelling RGCs and the expected TZ for their axonal projections in the lateral or medial contralateral SC, respectively. Bottom, dorsal view of a midbrain whole-mount depicting a normal TZ in the lateral SC from a WT mouse injected with DiI in the dorsal retina as verified in the flatmount (insert) and viewed using epifluorescence microscopy. ( b ) Top, example of a retina flatmount (insert) and SC whole mount from a WT mouse injected with DiI in the VT retina. Of 109 injected WT specimens analysed, only 3 formed one or more eTZs (3%). Bottom, the SC for each specimen that formed at least one eTZ had their eTZs and corresponding primary TZ outlined in the same colour. All outlines of the same genotype, in this case WT, were then superimposed on each other with the primary TZ positioned at the crosshairs of the compass as illustrated. ( c ) VT injected EphB2 lacZ/+ heterozygotes formed eTZs (arrows) in 7/22 SC analysed. ( d ) VT injected EphB2 lacZ/lacZ homozygotes formed eTZs (arrows) in 8/13 SC analysed. ( e ) Graphic summary of the percent of SC that formed eTZs in mice injected with DiI in the dorsal or VT retina. Dorsal injected: WT (1%, n =87), EphB2 +/− (15%, P =0.0437, n =13), EphB2 −/− (0%, n =3), EphB2 lacZ/+ (0%, n =35), and EphB2 lacZ/lacZ (0%, n =25). VT injected: WT (3%, n =109), EphB2 +/− (6%, n =16), EphB2 −/− (21%, P =0.0194, n =14), EphB2 lacZ/+ (32%, P =0.0001, n =22), and EphB2 lacZ/lacZ (62%, P <0.0001, n =13). FET compared mutant groups with WT mice. Statistical significance is denoted by asterisks: * P ≤0.05; ** P ≤0.01, and *** P ≤0.001. Scale bar, 500 μm. C, caudal; L, lateral; M, medial; R, rostral. Full size image EphB2 −/− protein-null single mutants and EphB2 lacZ/lacZ C-terminal truncation mutants [6] were used to determine the involvement of EphB2 and the contribution of its intracellular domain, respectively. Only 21% ( P =0.0194, Fisher's exact test [FET], n =14) of VT injected EphB2 −/− homozygotes and 6% ( n =16) of the EphB2 +/− heterozygotes formed 1-3 eTZs. In contrast, 62% ( P <0.0001, FET, n =13) of the EphB2 lacZ/lacZ homozygotes formed 1–4 eTZs and even 32% ( P =0.0049, FET, n =22) of the EphB2 lacZ/+ heterozygotes formed 1–3 eTZs ( Fig. 2c–e ). Whereas many eTZs were lateral to the primary TZ, RGC axons also terminated caudal relative to the primary TZ in several cases. The increased frequency of mapping errors in the EphB2 lacZ mice indicates a dominant-negative effect due to expression of the C-terminal truncated EphB2–β-gal fusion protein as seen in other studies [4] , [8] , [10] . Together, these data show that disruption of EphB2 forward signalling hinders the formation of a properly localized, single TZ in axons from the VT retina. EphB2 mutant SC that received focal injections of DiI into the dorsal retina did not significantly form any eTZs. Neither the EphB2 lacZ/+ ( n =35) or EphB2 lacZ/lacZ ( n =25) forward signalling mutants formed any eTZ and only 15% ( n =13) of the EphB2 +/− and 0% of the EphB2 −/− ( n =3) formed an eTZ ( Fig. 2e ), indicating EphB2 participates mainly in retinocollicular mapping of ventral RGC axons. EphB2 kinase activity is essential for VT axon mapping The data above using the EphB2 lacZ allele indicated a critical role for EphB2 forward signalling in retinocollicular mapping; however, it does not identify the specific intracellular signalling component responsible. Therefore, a variety of point mutations were analysed that disrupt either tyrosine kinase catalytic activity ( EphB2 K661R ), the ability to bind PDZ domain-containing proteins ( EphB2 ΔVEV ), or both catalytic activity and PDZ binding ( EphB2 K661RΔVEV ) [11] . VT RGC axons in 50% ( P <0.0001, FET, n =10) of the EphB2 K661R/K661R homozygotes and 21% ( P =0.0194, FET, n =14) of the EphB2 K661R/+ heterozygotes formed 1–2 eTZs lateral to the primary TZ ( Fig. 3a,b ). The penetrance of eTZs in the EphB2 K661R mutants was not significantly different from corresponding EphB2 lacZ mutants indicating the tyrosine kinase catalytic activity is the key component for EphB2 intracellular signalling required for VT axon retinocollicular mapping. 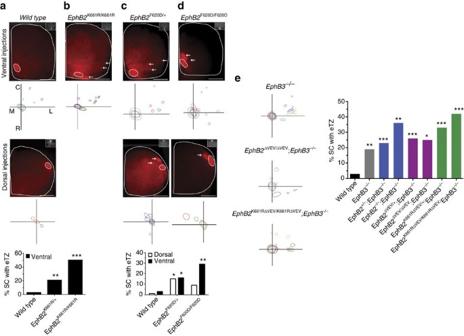Figure 3: EphB2 kinase activity is essential for topographic mapping of RGC axons from the VT retina. (a) Example of retinal flatmounts (inserts), SC whole mounts, and summary schematics of eTZs in WT specimens injected with DiI in the VT or dorsal retina. (b) VT injectedEphB2K661R/K661Rhomozygotes formed eTZs (arrows) in 5/10 SC analysed. Graphic summary of the percent of SC that formed eTZs in mice injected in the VT retina: WT (3%,n=109),EphB2K661R/+(21%,P=0.0194,n=14), andEphB2K661R/K661R(50%,P<0.0001,n=10). (c) VT injectedEphB2F620D/+heterozygotes formed eTZs (arrows) in 3/19 SC analysed and those injected in the dorsal retina formed eTZs in 4/26 SC. (d) VT injectedEphB2F620D/F620Dhomozygotes formed eTZs (arrows) in 5/17 SC analysed and those injected in the dorsal retina formed eTZs in 2/22 SC. Graphic summary of the percent of SC that formed eTZs in mice injected in the dorsal or VT retina. Dorsal injected: WT (1%,n=87),EphB2F620D/+(15%,P=0.0257,n=26), andEphB2F620D/F620D(9%,n=22). VT injected: WT (3%,n=109),EphB2F620D/+(16%,P=0.042,n=19), andEphB2F620D/F620D(29%,P=0.0011,n=17). (e) Schematic of eTZs fromEphB3−/−single mutants andEphB2ΔVEV/ΔVEV;EphB3−/−andEphB2K661RΔVEV/K661RΔVEV;EphB3−/−compound mutants injected with DiI into the VT retina. VT injectedEphB3−/−homozygotes formed eTZs in 9/48 SC,EphB2ΔVEV/ΔVEV;EphB3−/−compound mutants formed eTZ in 3/12 SC, andEphB2K661RΔVEV/K661RΔVEV;EphB3−/−compound mutants formed eTZ in 8/19 SC. Graphic summary of the percent of SC that formed eTZs in mice injected with DiI into the VT retina: WT (3%,n=109),EphB3−/−(19%,P=0.0013,n=48),EphB2+/−;EphB3−/−(23%,P=0.0001,n=48),EphB2−/−;EphB3−/−(36%,P=0.0012,n=11),EphB2ΔVEV/+;EphB3−/−(26%,P=0.0009,n=23),EphB2ΔVEV/ΔVEV;EphB3−/−(25%,P=0.0128,n=12),EphB2K661RΔVEV/+;EphB3−/−(33%,P<0.0001,n=24), andEphB2K661RΔVEV/K661RΔVEV;EphB3−/−(42%,P<0.0001,n=19). FET compared mutant groups to WT mice. Statistical significance is denoted by asterisks: *P≤0.05; **P≤0.01, and ***P≤0.001. Scale bar, 500 μm. C, caudal; L, lateral; M, medial; R, rostral. Figure 3: EphB2 kinase activity is essential for topographic mapping of RGC axons from the VT retina. ( a ) Example of retinal flatmounts (inserts), SC whole mounts, and summary schematics of eTZs in WT specimens injected with DiI in the VT or dorsal retina. ( b ) VT injected EphB2 K661R/K661R homozygotes formed eTZs (arrows) in 5/10 SC analysed. Graphic summary of the percent of SC that formed eTZs in mice injected in the VT retina: WT (3%, n =109), EphB2 K661R/+ (21%, P =0.0194, n =14), and EphB2 K661R/K661R (50%, P <0.0001, n =10). ( c ) VT injected EphB2 F620D/+ heterozygotes formed eTZs (arrows) in 3/19 SC analysed and those injected in the dorsal retina formed eTZs in 4/26 SC. ( d ) VT injected EphB2 F620D/F620D homozygotes formed eTZs (arrows) in 5/17 SC analysed and those injected in the dorsal retina formed eTZs in 2/22 SC. Graphic summary of the percent of SC that formed eTZs in mice injected in the dorsal or VT retina. Dorsal injected: WT (1%, n =87), EphB2 F620D/+ (15%, P =0.0257, n =26), and EphB2 F620D/F620D (9%, n =22). VT injected: WT (3%, n =109), EphB2 F620D/+ (16%, P =0.042, n =19), and EphB2 F620D/F620D (29%, P =0.0011, n =17). ( e ) Schematic of eTZs from EphB3 −/− single mutants and EphB2 ΔVEV/ΔVEV ;EphB3 −/− and EphB2 K661RΔVEV/K661RΔVEV ;EphB3 −/− compound mutants injected with DiI into the VT retina. VT injected EphB3 −/− homozygotes formed eTZs in 9/48 SC, EphB2 ΔVEV/ΔVEV ;EphB3 −/− compound mutants formed eTZ in 3/12 SC, and EphB2 K661RΔVEV/K661RΔVEV ;EphB3 −/− compound mutants formed eTZ in 8/19 SC. Graphic summary of the percent of SC that formed eTZs in mice injected with DiI into the VT retina: WT (3%, n =109), EphB3 −/− (19%, P =0.0013, n =48), EphB2 +/− ;EphB3 −/− (23%, P =0.0001, n =48), EphB2 −/− ;EphB3 −/− (36%, P =0.0012, n =11), EphB2 ΔVEV/+ ;EphB3 −/− (26%, P =0.0009, n =23), EphB2 ΔVEV/ΔVEV ;EphB3 −/− (25%, P =0.0128, n =12), EphB2 K661RΔVEV/+ ;EphB3 −/− (33%, P <0.0001, n =24), and EphB2 K661RΔVEV/K661RΔVEV ;EphB3 −/− (42%, P <0.0001, n =19). FET compared mutant groups to WT mice. Statistical significance is denoted by asterisks: * P ≤0.05; ** P ≤0.01, and *** P ≤0.001. Scale bar, 500 μm. C, caudal; L, lateral; M, medial; R, rostral. Full size image The involvement of EphB2 tyrosine kinase activity was also examined using kinase overactive EphB2 F620D mutants that contains a point mutation in the catalytic domain rendering EphB2 constitutively active, independent of ligand binding [12] . While 16% ( P =0.042, FET, n =19) of VT injected EphB2 F620D/+ heterozygotes formed 1–3 lateral eTZs, 29% ( P =0.0011, FET, n =17) of the corresponding EphB2 F620D/F620D homozygotes formed 1–2 lateral or caudal eTZs ( Fig. 3c,d ). Of the specimens injected with DiI into the dorsal retina, 15% ( P =0.0257, FET, n =26) of the EphB2 F620D/+ heterozygotes and 9% ( n =22) of EphB2 F620D/F620D homozygotes formed 1–2 eTZs medial to the primary TZ ( Fig. 3c,d ). Combined, these data suggest that both ventral and dorsal RGC axons are somewhat affected by an overactive EphB2 catalytic domain, which is consistent with the robust ventral EphB2 expression and low, although detectable, level of EphB2 expression in the dorsal retina. The contribution of the EphB2 PDZ binding motif to retinocollicular mapping of VT axons was also examined in EphB2 ΔVEV/ΔVEV mutants in the background of the EphB3 −/− protein-null mutant and was found not to participate in TZ formation, whereas the corresponding EphB2 K661RΔVEV/K661RΔVEV ; EphB3 −/− compound mutants showed no extra defects over what was found for the EphB2 K661R/K661R kinase-dead single mutants ( Fig. 3e ). EphB1 forward signalling is also utilized for VT axon mapping Previous studies have not looked at potential roles of the EphB1 receptor tyrosine kinase in retinocollicular mapping, even though it is expressed in the visual system ( Fig. 1b ) and has been documented to mediate the repulsion of VT RGC axons at the optic chiasm to form ipsilateral projections [5] . Therefore, VT and dorsal RGC axons were labelled with DiI in EphB1 −/− protein-null mutants. Whereas dorsal RGC axons terminated normally to a well-defined TZ, the VT axons in EphB1 −/− homozygotes exhibited a highly penetrant mapping defect in which 65% ( P <0.0001, FET, n =20) of the SC showed 1–3 eTZs ( Fig. 4a,b ). Even 38% ( P =0.0003, FET, n =13) of the VT-labelled EphB1 +/− heterozygotes formed 1–3 eTZs, indicating a strong dosage effect. These eTZs tended to form lateral relative to the primary TZ. Additionally, it was often noted that the primary TZ in the mutants was not compact like that observed in WT, and, in one case, a distinct primary TZ was not visible. 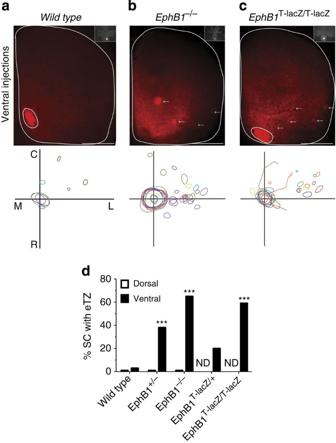Figure 4: EphB1 forward signalling is important for topographic mapping of axons from the VT retina. (a) Example of retinal flatmount (insert), SC whole mount, and summary schematic of eTZs in WT specimens injected with DiI in the VT retina. (b) VT injectedEphB1−/−homozygotes formed eTZs (arrows) in 13/20 SC analysed. (c) VT injectedEphB1T-lacZ/T-lacZhomozygotes formed eTZs (arrows) in 10/17 SC analysed. (d) Graphic summary of the percent of SC that formed eTZs in mice injected in the dorsal or VT retina. Dorsal injected: WT (1%,n=87),EphB1+/−(0%,n=15), andEphB1−/−(0%,n=13). VT injected: WT (3%,n=109),EphB1+/−(38%,P=0.0003,n=13),EphB1−/−(65%,P<0.0001,n=20),EphB1T-lacZ/+(20%,n=5), andEphB1T-lacZ/T-lacZ(59%,P<0.0001,n=17). ND, not done. FET compared mutant groups with WT mice. Statistical significance is denoted by asterisks: *P≤0.05; **P≤0.01, and ***P≤0.001. Scale bar, 500 μm. C, caudal; L, lateral; M, medial; R, rostral. Figure 4: EphB1 forward signalling is important for topographic mapping of axons from the VT retina. ( a ) Example of retinal flatmount (insert), SC whole mount, and summary schematic of eTZs in WT specimens injected with DiI in the VT retina. ( b ) VT injected EphB1 −/− homozygotes formed eTZs (arrows) in 13/20 SC analysed. ( c ) VT injected EphB1 T-lacZ/T-lacZ homozygotes formed eTZs (arrows) in 10/17 SC analysed. ( d ) Graphic summary of the percent of SC that formed eTZs in mice injected in the dorsal or VT retina. Dorsal injected: WT (1%, n =87), EphB1 +/− (0%, n =15), and EphB1 −/− (0%, n =13). VT injected: WT (3%, n =109), EphB1 +/− (38%, P =0.0003, n =13), EphB1 −/− (65%, P <0.0001, n =20), EphB1 T-lacZ/+ (20%, n =5), and EphB1 T-lacZ/T-lacZ (59%, P <0.0001, n =17). ND, not done. FET compared mutant groups with WT mice. Statistical significance is denoted by asterisks: * P ≤0.05; ** P ≤0.01, and *** P ≤0.001. Scale bar, 500 μm. C, caudal; L, lateral; M, medial; R, rostral. Full size image To determine whether forward signalling mediated by the EphB1 intracellular domain is important, EphB1 T-lacZ mutant mice expressing the C-terminal truncated EphB1–β-gal fusion protein described above were analysed. The data showed that 59% ( P <0.0001, FET, n =17) of the EphB1 T-lacZ/T-lacZ homozygotes and 20% ( P =ns, FET, n =5) of the EphB1 T-lacZ/+ heterozygotes formed 1–3 eTZs usually lateral to the primary TZ following DiI injection into the VT retina ( Fig. 4c,d ). Like EphB2, these results indicate that forward signalling mediated by the EphB1 intracellular domain is required for retinocollicular mapping of VT RGC axons. Synergistic role for EphB1 and EphB2 in VT axon mapping To determine whether EphB1 and EphB2 work together to mediate retinocollicular mapping, DiI was used to trace RGC axons in EphB1 ; EphB2 compound mutants. The EphB1 − protein-null allele was combined with either EphB2 − protein-null, eliminating both forward and reverse signalling, or the EphB2 lacZ allele, eliminating only EphB2 forward signalling. Following labelling of VT RGC axons, 100% of the EphB1 −/− ;EphB2 +/− ( P <0.0001, FET, n =12,) and EphB1 −/− ;EphB2 −/− ( P <0.0001, FET, n =7) SC analysed exhibited 1–5 eTZs that localized caudal, lateral, and lateral–caudal relative to the primary TZ ( Fig. 5a,b ). These mutants also exhibited an increase in stray axonal projections, and the primary TZ was often not fully compact, appearing diffused, compared with WT. The complete 100% penetrance and severity of the mapping defect indicates these molecules work synergistically to control the targeting of VT RGC axons within the SC. 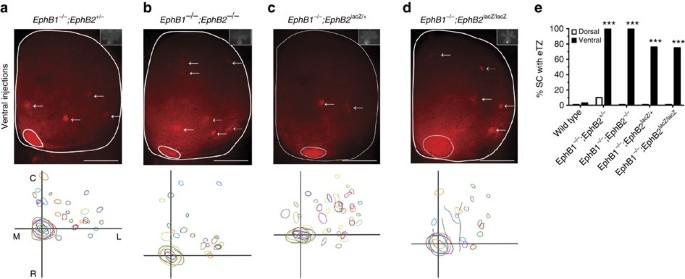Figure 5: Synergistic role for both EphB1 and EphB2 in topographic mapping of axons from the VT retina. (a) VT injectedEphB1−/−;EphB2+/−compound mutants formed eTZs (arrows) in 12/12 SC analysed. (b) VT injectedEphB1−/−;EphB2−/−compound homozygotes formed eTZs (arrows) in 7/7 SC analysed. (c) VT injectedEphB1−/−;EphB2lacZ/+compound mutants formed eTZs (arrows) in 16/21 SC analysed. (d) VT injectedEphB1−/−;EphB2lacZ/lacZcompound homozygotes formed eTZs (arrows) in 6/8 SC analysed. (e) Graphic summary of the percent of SC that formed eTZs in mice injected in the dorsal or VT retina. Dorsal injected: WT (1%,n=87),EphB1−/−;EphB2+/−(10%,n=10),EphB1−/−;EphB2−/−(0%,n=7),EphB1−/−;EphB1lacZ/+(0%,n=11), andEphB1−/−;EphB1lacZ/lacZ(0%,n=9). VT injected: WT (3%,n=109),EphB1−/−;EphB2+/−(100%,P<0.0001,n=12),EphB1−/−;EphB2−/−(100%,P<0.0001,n=7),EphB1−/−;EphB1lacZ/+(76%,P<0.0001,n=21), andEphB1−/−;EphB1lacZ/lacZ(75%,P<0.0001,n=8). FET compared mutant groups with WT mice. Statistical significance is denoted by asterisks: *P≤0.05; **P≤0.01, and ***P≤0.001. Scale bar, 500 μm. C, caudal; L, lateral; M, medial; R, rostral. Figure 5: Synergistic role for both EphB1 and EphB2 in topographic mapping of axons from the VT retina. ( a ) VT injected EphB1 −/− ; EphB2 +/− compound mutants formed eTZs (arrows) in 12/12 SC analysed. ( b ) VT injected EphB1 −/− ; EphB2 −/− compound homozygotes formed eTZs (arrows) in 7/7 SC analysed. ( c ) VT injected EphB1 −/− ; EphB2 lacZ/+ compound mutants formed eTZs (arrows) in 16/21 SC analysed. ( d ) VT injected EphB1 −/− ; EphB2 lacZ/lacZ compound homozygotes formed eTZs (arrows) in 6/8 SC analysed. ( e ) Graphic summary of the percent of SC that formed eTZs in mice injected in the dorsal or VT retina. Dorsal injected: WT (1%, n =87), EphB1 −/− ; EphB2 +/− (10%, n =10), EphB1 −/− ;EphB2 −/− (0%, n =7), EphB1 −/− ;EphB1 lacZ/+ (0%, n =11), and EphB1 −/− ;EphB1 lacZ/lacZ (0%, n =9). VT injected: WT (3%, n =109), EphB1 −/− ;EphB2 +/− (100%, P <0.0001, n =12), EphB1 −/− ;EphB2 −/− (100%, P <0.0001, n =7), EphB1 −/− ;EphB1 lacZ/+ (76%, P <0.0001, n =21), and EphB1 −/− ;EphB1 lacZ/lacZ (75%, P <0.0001, n =8). FET compared mutant groups with WT mice. Statistical significance is denoted by asterisks: * P ≤0.05; ** P ≤0.01, and *** P ≤0.001. Scale bar, 500 μm. C, caudal; L, lateral; M, medial; R, rostral. Full size image Likewise, compound mutant mice carrying the EphB1 − and EphB2 lacZ alleles had near-full penetrance of mapping defects. Seventy-six percent ( P <0.0001, FET, n =21) of the EphB1 −/− ;EphB2 lacZ/+ and 75% ( P <0.0001, FET, n =8) of the EphB1 −/− ;EphB2 lacZ/lacZ mutant SC formed 1–6 eTZs that localized lateral, caudal, and lateral–caudal directions relative to the primary TZ ( Fig. 5c,d ). The primary TZs were also often not compact, and exhibited stray axonal projections. Dorsal RGC axons formed no eTZs ( n =7) in the EphB1 −/− : EphB2 −/− compound nulls, and only 1 ( n =10) of the EphB1 −/− ;EphB2 +/− SC analysed did so ( Fig. 5e ). Together, these data demonstrate the vital and specific role for EphB1/EphB2-mediated forward signalling in VT RGC axons. Ephrin-B1 mediates VT RGC axon mapping within the SC Elevated ephrin-B1 expression at the midline of the SC or optic tectum (OT) suggests the potential role of ephrin-B1 acting as a ligand to mediate VT RGC axon interstitial branching and termination in the medial SC [4] , [13] , [14] , [15] , [16] . In chick and Xenopus laevis , ephrin-B1 mRNA is expressed along the midline of OT [13] , [14] . In the mouse SC, ephrin-B1 protein is found in a high medial/low lateral gradient in the superficial layer at P0 (ref. 4 ), though recent analysis described ephrin-B1 uniformly expressed at P2 in the superficial and deeper layers of the SC [15] . Demonstrating the important role for this expression, ephrin-B1 ectopic expression in the chick OT disrupted the direction of ventral RGC axon interstitial branching resulting in ectopic axon terminations [16] . To determine whether the absence of ephrin-B1 expression affects retinocollicular mapping, we analysed germ-line protein-null mutant mice that carried a deletion in the X-linked ephrin-B1 gene [17] . DiI-labelled dorsal RGC axons from ephrin-B1 +/− ( n =4) and ephrin-B1 −/y ( n =17) mice had no retinocollicular mapping errors. However, VT RGC axons formed 1 eTZ in 25% ( P =0.0128, FET, n =12) of the ephrin-B1 −/y hemizygous male mice and in 33% ( P =0.0213, FET, n =6) of the ephrin-B1 +/− female mice, that were small and either caudal or lateral to the primary TZ ( Fig. 6 ). These data indicate that ephrin-B1 expressed in the SC midline acts as ligand to mediate EphB1/EphB2 forward signal-driven VT RGC axon retinocollicular mapping, although the incomplete penetrance of the defect suggests that other ephrin molecules likely participate. 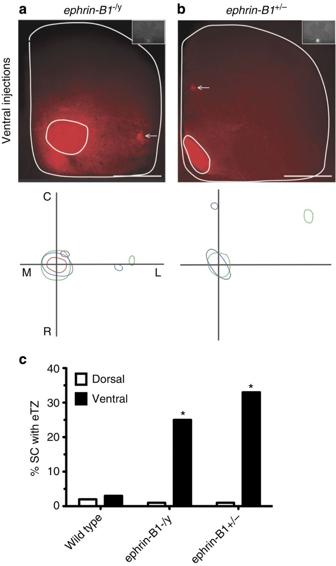Figure 6: Ephrin-B1 mediates topographic mapping of axons from the VT retina. (a) VT injectedephrin-B1-/yhemizygous males formed eTZs (arrows) in 3/12 SC analysed. (b) VT injectedephrin-B1+/−heterozygous females formed eTZs (arrows) in 2/6 SC analysed. (c) Graphic summary of the percent of SC that formed eTZs in mice injected in the dorsal or VT retina. Dorsal injected: WT (1%,n=87),ephrin-B1−/y(0%,n=17), andephrin-B1+/−(0%,n=4). VT injected: WT (3%,n=109),ephrin-B1−/y(25%,P=0.0128,n=12), andephrin-B1+/−(33%,P=0.0213,n=6). FET compared mutant groups with WT mice. Statistical significance is denoted by asterisks: *P≤0.05; **P≤0.01, and ***P≤0.001. Scale bar, 500 μm. C, caudal; L, lateral; M, medial; R, rostral. Figure 6: Ephrin-B1 mediates topographic mapping of axons from the VT retina. ( a ) VT injected ephrin-B1 -/y hemizygous males formed eTZs (arrows) in 3/12 SC analysed. ( b ) VT injected ephrin-B1 +/− heterozygous females formed eTZs (arrows) in 2/6 SC analysed. ( c ) Graphic summary of the percent of SC that formed eTZs in mice injected in the dorsal or VT retina. Dorsal injected: WT (1%, n =87), ephrin-B1 −/y (0%, n =17), and ephrin-B1 +/− (0%, n =4). VT injected: WT (3%, n =109), ephrin-B1 −/y (25%, P =0.0128, n =12), and ephrin-B1 +/− (33%, P =0.0213, n =6). FET compared mutant groups with WT mice. Statistical significance is denoted by asterisks: * P ≤0.05; ** P ≤0.01, and *** P ≤0.001. Scale bar, 500 μm. C, caudal; L, lateral; M, medial; R, rostral. Full size image Dorsal and VT axons require ephrin-B2 reverse signalling To study roles for ephrin-B2-mediated reverse signalling in the mouse, we analysed ephrin-B2 lacZ mutants that express a C-terminal, intracellular truncated ephrin-B2–β-gal fusion protein. While unable to transduce reverse signals, the ephrin-B2–β-gal fusion protein can still act as a ligand to stimulate forward signalling [18] . Because ephrin-B2 lacZ/lacZ homozygotes do not survive after birth, this allele was combined with a new mutation described here, ephrin-B2 6YFΔV . This ephrin-B2 6YFΔV allele carries point mutations in the exon that encodes the intracellular cytoplasmic tail that change the 6 tyrosine residues into phenylalanines and also deletes the C-terminal valine residue ( Supplementary Fig. S1 ). As a result, this mutation expresses a protein that is properly localized to the cell surface ( Supplementary Fig. S2 ) but is unable to become tyrosine phosphorylated or interact with either SH2 or PDZ domain-containing downstream signalling proteins. Previous studies have shown that similar mutations in ephrin-B1 and ephrin-B3 express proteins that lose their ability to transduce canonical ephrin-B reverse signals but maintain their ability to act as ligands to transduce forward signals in adjacent EphB-expressing cells [19] , [20] . Ephrin-B2 lacZ/+ males were mated to ephrin-B2 6YFΔV/+ females and the resulting offspring were analysed by DiI labelling of dorsal RGC axons. We observed the formation of 1–2 eTZs medial or medial-rostral to the primary TZ in 11% ( P =0.0442, FET, n =28) of ephrin-B2 6YFΔV/+ SC, 8% ( P =ns, FET, n =26) of the ephrin-B2 lacZ/+ SC, and 27% ( P =0.0015, FET, n =15) of the ephrin-B2 lacZ/6YFΔV SC ( Fig. 7 ). This demonstrates that ephrin-B2 reverse signalling is required for dorsal RGC axon retinocollicular mapping. 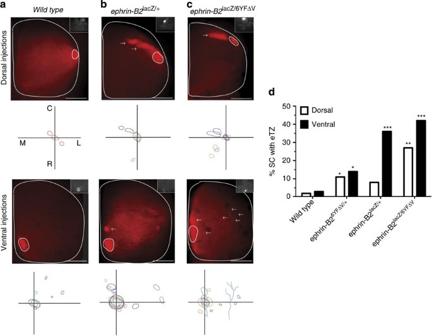Figure 7: Dorsal and VT RGC axons require ephrin-B2 reverse signalling for topographic mapping. (a) Example of retinal flatmounts (inserts), SC whole mounts, and summary schematics of eTZs in WT specimens injected with DiI in the VT or dorsal retina. (b) Dorsal injectedephrin-B2lacZ/+heterozygotes formed eTZs (arrows) in 2/26 SC analysed and those injected in the VT retina formed eTZs in 8/22 SC. (c) Dorsal injectedephrin-B2lacZ/6YFΔVmutants formed eTZs (arrows) in 4/15 SC analysed and those injected in the VT retina formed eTZs in 5/12 SC. (d) Graphic summary of the percent of SC that formed eTZs in mice injected in the dorsal or VT retina. Dorsal injected: WT (1%,n=87),ephrin-B26YFΔV/+(11%,P=0.0442,n=28),ephrin-B2lacZ/+(8%,n=26), andephrin-B2lacZ/6YFΔV(27%,P=0.0015,n=15). VT injected: WT (3%,n=109),ephrin-B26YFΔV/+(14%,P=0.0105,n=49),ephrin-B2lacZ/+(36%,P<0.0001,n=22), andephrin-B2lacZ/6YFΔV(42%,P=0.0002,n=12). FET compared mutant groups with WT mice. Statistical significance is denoted by asterisks: *P≤0.05; **P≤0.01, and ***P≤0.001. Scale bar, 500 μm. C, caudal; L, lateral; M, medial; R, rostral. Figure 7: Dorsal and VT RGC axons require ephrin-B2 reverse signalling for topographic mapping. ( a ) Example of retinal flatmounts (inserts), SC whole mounts, and summary schematics of eTZs in WT specimens injected with DiI in the VT or dorsal retina. ( b ) Dorsal injected ephrin-B2 lacZ/+ heterozygotes formed eTZs (arrows) in 2/26 SC analysed and those injected in the VT retina formed eTZs in 8/22 SC. ( c ) Dorsal injected ephrin-B2 lacZ/6YFΔV mutants formed eTZs (arrows) in 4/15 SC analysed and those injected in the VT retina formed eTZs in 5/12 SC. ( d ) Graphic summary of the percent of SC that formed eTZs in mice injected in the dorsal or VT retina. Dorsal injected: WT (1%, n =87), ephrin-B2 6YFΔV/+ (11%, P =0.0442, n =28), ephrin-B2 lacZ/+ (8%, n =26), and ephrin-B2 lacZ/6YFΔV (27%, P =0.0015, n =15). VT injected: WT (3%, n =109), ephrin-B2 6YFΔV/+ (14%, P =0.0105, n =49), ephrin-B2 lacZ/+ (36%, P <0.0001, n =22), and ephrin-B2 lacZ/6YFΔV (42%, P =0.0002, n =12). FET compared mutant groups with WT mice. Statistical significance is denoted by asterisks: * P ≤0.05; ** P ≤0.01, and *** P ≤0.001. Scale bar, 500 μm. C, caudal; L, lateral; M, medial; R, rostral. Full size image Whereas the gradient of ephrin-B2 expression is at an obviously lower level in the ventral retina compared with the dorsal retina, its ventral expression is evident at E17.5 and becomes more pronounced during the first postnatal week as observed at P0 and P8 ( Fig. 1c ). This indicates ephrin-B2 may also participate in ventral RGC axon retinocollicular mapping. Indeed, DiI tracing of VT RGC axons indicated 1–2 eTZs lateral or caudal to the primary TZ in 14% ( P =0.0105, FET, n =49) of the ephrin-B2 6YFΔV/+ SC and 36% ( P <0.0001, FET, n =22) of the ephrin-B2 lacZ/+ SC ( Fig. 7 ). The severity of the mapping defect increased in ephrin-B2 lacZ/6YFΔV SC in which 42% ( P =0.0002, FET, n =12) of the SC formed 1–3 eTZs lateral, caudal, and rostral relative to the primary TZ ( Fig. 7 ). These data indicate a previously unanticipated role for ephrin-B2 reverse signalling in VT RGC retinocollicular mapping. As illustrated in the schematic ( Fig. 8 ), we determined that EphB2 tyrosine kinase catalytic activity and EphB1 forward signalling are required for VT RGC axon retinocollicular mapping and that ephrin-B1 is their likely ligand. We further show that ephrin-B2 acts as a receptor to transduce reverse signals necessary for both dorsal and ventral RGC axon mapping. 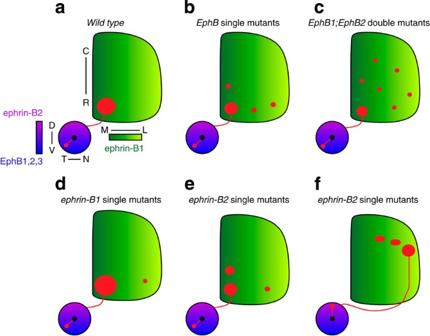Figure 8: Summary of mapping errors inEphBandephrin-Bmutants. (a) VT RGC axons in WT terminate in the medial SC and form a single compact TZ by P8. Red illustrates the subgroup of RGC axons labelled by DiI and their termination in the SC. Blue represents the EphB high ventral/low dorsal gradient in the retina, whereas the purple represents the high dorsal/low ventral ephrin-B2 gradient. Green shows the high medial expression of ephrin-B1 in the SC. C, caudal; D, dorsal; L, lateral; M, medial; R, rostral; V, ventral. (b) Subset of VT RGC axons inEphBsingle protein-null and forward signalling mutants formed 1–3 eTZs lateral and sometimes caudal to the primary TZ. (c) Subset of VT RGC axons inEphB1;EphB2compound protein-null and forward signalling mutants formed 1–6 eTZs lateral, caudal, and caudal–lateral to the primary TZ. The primary TZ was often reduced, dispersed, and/or projected stray axons. (d) Subset of VT RGC axons inephrin-B1protein-null mutants formed 1 eTZ lateral to the primary TZ. The primary TZ was dispersed in these mutants. (e) Subset of VT RGC axons inephrin-B2reverse signalling mutants formed 1–2 eTZ caudal and sometimes lateral to the primary TZ. (f) Subset of dorsal RGC axons inephrin-B2reverse signalling mutants formed 1-2 eTZ medial to the primary TZ. Figure 8: Summary of mapping errors in EphB and ephrin-B mutants. ( a ) VT RGC axons in WT terminate in the medial SC and form a single compact TZ by P8. Red illustrates the subgroup of RGC axons labelled by DiI and their termination in the SC. Blue represents the EphB high ventral/low dorsal gradient in the retina, whereas the purple represents the high dorsal/low ventral ephrin-B2 gradient. Green shows the high medial expression of ephrin-B1 in the SC. C, caudal; D, dorsal; L, lateral; M, medial; R, rostral; V, ventral. ( b ) Subset of VT RGC axons in EphB single protein-null and forward signalling mutants formed 1–3 eTZs lateral and sometimes caudal to the primary TZ. ( c ) Subset of VT RGC axons in EphB1 ; EphB2 compound protein-null and forward signalling mutants formed 1–6 eTZs lateral, caudal, and caudal–lateral to the primary TZ. The primary TZ was often reduced, dispersed, and/or projected stray axons. ( d ) Subset of VT RGC axons in ephrin-B1 protein-null mutants formed 1 eTZ lateral to the primary TZ. The primary TZ was dispersed in these mutants. ( e ) Subset of VT RGC axons in ephrin-B2 reverse signalling mutants formed 1–2 eTZ caudal and sometimes lateral to the primary TZ. ( f ) Subset of dorsal RGC axons in ephrin-B2 reverse signalling mutants formed 1-2 eTZ medial to the primary TZ. Full size image Fifty per cent or greater of the EphB1 −/− , EphB1 T-lacZ/T-lacZ , EphB2 K661R/K661R , and EphB2 lacZ/lacZ single mutant mice exhibited mapping defects, thus, demonstrating that EphB1 and EphB2 each have a critical role. However, when we analysed VT-labelled axons in EphB1 −/− ;EphB2 −/− mutants, the mapping defect reached complete penetrance and had severely disrupted retinocollicular maps indicating EphB1/EphB2-mediated forward signalling is vital. A role for the EphB receptor extracellular domain in stimulating reverse signalling is also evident. Whereas EphB1 −/− ;EphB2 lacZ/lacZ and EphB1 −/− ;EphB2 lacZ/+ mutants exhibited mapping defects as severe as those observed in the EphB1 −/− ;EphB2 −/− mutants, the penetrance decreased from 100% to 75%. Furthermore, the EphB2 −/− mutants displayed mapping defects that were less penetrant compared with the EphB2 lacZ/lacZ and EphB2 K661R/K661R mutants, whereas the EphB1 −/− and EphB1 T-lacZ/T-lacZ shared similar levels of penetrance. The presence of the EphB2 extracellular domain in the EphB2 lacZ/lacZ and EphB2 K661R/K661R mutants may disrupt the balance between reverse and forward signalling whereas the lack of EphB2 in EphB2 −/− mutants may result in an overall decrease in both forward and reverse signalling rather than an imbalance. The extracellular domain of EphB1 may not be essential so that elimination of EphB1 in the EphB1 −/− mutants results in disruption of only forward signalling resulting in an imbalance between forward and reverse signalling. Another interesting observation is that the loss of kinase activity only affects VT axons, while the kinase-overactive gain-of-function EphB2 F620D point mutant has both ventral and dorsal axons disrupted. EphB2 is expressed in the dorsal retina, albeit at relatively lower levels than in the ventral retina. Excessive unregulated kinase activity in the gain-of-function may have a much stronger effect in dorsal axons than loss of kinase activity, and this imbalance in signalling may cause them to behave more like VT axons leading to abnormal targeting. Whereas other studies have highlighted the role of EphB3 using EphB2;EphB3 compound mutants [4] , we evaluated roles for EphB1, EphB2, and EphB3 individually and in compound mutants. The VT RGC axons in EphB2 −/− and EphB3 −/− single mutants formed eTZs in about 20% of the SC whereas EphB2 −/− ; EphB3 −/− mutants formed eTZs in about 36% of the SC ( Figs 2 and 3 ). Although these data indicate that EphB3 is important in ventral RGC axon retinocollicular mapping, the EphB2 −/− ; EphB3 −/− mutants did not have the same severity or 100% penetrance as the EphB1 −/− ; EphB2 −/− mutants. VT RGC axons expressing high levels of EphB receptors target into the medial-rostral SC that expresses ephrin-B1. As hypothesized in other studies [4] and examined in the chick [16] , ephrin-B1 likely attracts RGC axon interstitial branches to the midline. This attraction is likely balanced by repulsion to the midline mediated by Wnt–Ryk signalling [3] . Our data is the first to show a mapping defect in ephrin-B1 mutant mice that supports this hypothesis, although surprisingly ephrin-B1 -deleted mutants do not disrupt retinocollicular mapping to the extent that the EphB1;EphB2 compound mutants do, indicating ephrin-B1 is not the sole ligand. Ephrin-B2 reverse signalling mutants not only disrupted dorsal RGC axon mapping, as predicted by its robust dorsal expression pattern, but also VT RGC axons. Dorsal RGC axons lacking ephrin-B2 reverse signalling still express EphB receptors, therefore, EphB forward signalling may become the dominant signalling mechanism resulting in too much attraction to the midline thus eTZs that form medial to the primary TZ. VT RGC axons lacking ephrin-B2 reverse signalling seem to form more eTZs along the rostrocaudal axis as well as lateral to the primary TZ, indicating that the lack of ephrin-B2 reverse signalling disrupts VT RGC axon targeting to the rostral-medial SC. Mediators for dorsal RGC axons in mice have not been found previously, although other studies show that ephrin-B2 reverse signalling is important for retinotopic mapping. In Xenopus laevis , ephrin-B2 mRNA is expressed in a high dorsal/low ventral gradient in the retina and along the midline of the OT [14] . Ectopic expression of a dominant-negative ephrin-B2 cytoplasmic tail deleted mutant in either the dorsal or ventral retina resulted in RGC axon targeting errors in the OT. Whereas this study in Xenopus and ours in mice show ephrin-B2 reverse signalling is important for dorsoventral RGC axon retinocollicular mapping, the ligand that ephrin-B2 interacts within the SC remains unknown. As the EphB1 and EphB2 single and compound null mutants showed no significant defect in dorsal RGC axon targeting, the data indicates these two Eph molecules are not acting as the principal ligands here to stimulate reverse signalling. While we identified ephrin-B1 as a ligand for VT axons, other unknown ligands must be present to explain the penetrance of defects observed in the EphB and ephrin-B2 mutants. In addition, as mentioned above, no ligand that stimulates reverse signalling in dorsal RGC axons has been identified in the SC. One possibility is that receptor and ligands co-expressed on RGC axons interact in cis with each other and promote interstitial branch extension in the SC, or perhaps interact with Ephs and ephrins localized on adjacent axons. Another possibility is that EphB/ephrin-B2 expressed on the RGC axons interact with EphA/ephrin-A expressed in the SC. The Eph and ephrin molecules generally interact within their own class, however some interclass promiscuity exists. Both EphA4 and EphB2 bind to ephrin-B1/2/3 and ephrin-A5, as visualized by crystal structures of EphB2:ephrin-A5 and EphA4:ephrin-B2 (refs 21 , 22 , 23 ). Ephrin-A5 has a high caudal/low rostral gradient expression in the SC and is critical for axon pruning of the initial overshoot of the RGC axons past their proper TZ during the first postnatal week. Considering the established activation of EphB2 forward signalling by ephrin-A5 (ref. 21 ), VT RGC axons may be responding to the ephrin-A5 gradient. Likewise, ephrin-B2 may interact with EphA4, which is expressed in the SC [24] . Supporting this hypothesis is the localization of eTZs along the rostrocaudal axis observed in VT axons of EphB and ephrin-B2 mutants. These interactions may contribute to the formation of rostral and caudal eTZs relative to the primary TZ in EphB and ephrin-B mutant SC as well as why the deletion of ephrin-B1 does not result in a fully penetrant defect. Mice Generation of CD1 background EphB and ephrin-B mutant mice and genotyping by PCR have been described previously for the following alleles used: EphB1 − (ref. 5 ), EphB1 lacZ (ref. 5 ), EphB2 − (ref. 6 ), EphB2 lacZ (ref. 6 ), EphB2 ΔVEV (ref. 11 ), EphB2 K661R (ref. 11 ), EphB2 K661RΔVEV (ref. 11 ), EphB2 F620D (ref. 12 ), EphB3 − (ref. 25 ), ephrin-B1 loxP (ref. 17 ), ephrin-B2 lacZ (ref. 8 ). The EphB1 T-lacZ mutation inserts bacterial lacZ sequence in frame within exon 9 immediately following the codon corresponding to murine EphB1 amino acid #578 (ref. 7 ). The ephrin-B1 − allele was generated by crossing the ephrin-B1 loxP conditional allele to a transgenic mouse that expresses Cre recombinase in the germline. All experiments involving mice were carried out in accordance with the US National Institutes of Health Guide for the Care and Use of Animals under an Institutional Animal Care and Use Committee-approved protocol and Association for Assessment and Accreditation of Laboratory Animal Care-approved facility at the University of Texas Southwestern Medical Center. Approximately equal numbers of males and females were used in the analysis without any differences noted. Generation of the ephrin-B2 6YFΔV mutation To construct the targeting vector, a bacterial artificial chromosome contig encompassing genomic DNA surrounding ephrin-B2 exon 5, which encodes the entire intracellular domain of ephrinB2, was first assembled in pBeloBAC11 from genomic mouse DNA by combining lambda phage clones EB2.9 and EB2.22 using recombineering in Escherichia coli strain EL 250 (ref. 26 ). Using a pL452-based mini-targeting vector that contained a positive selection neo cassette, a WT 300 bp 5′-arm of exon 5, and a 1,200 bp 3′-arm containing base pair modifications corresponding to the desired 6YFΔV mutations (Y255F, Y307F, Y314F, Y319F, Y333F, Y334F, and Δ336 V) was recombined with endogenous ephrin-B2 sequence. A targeting vector was retrieved into pL254 (a modified form of pL253 with a 3′ TK and extra DT-A negative selection cassette and an AscI restriction enzyme site for linearization). R1 embryonic stem cells [27] were electroporated, and colonies were screened by Southern blotting. Germline transmission was obtained from chimeric mice generated by blastocyst injection. The loxP floxed neo cassette was subsequently deleted in the mouse by crossing to a germline expressing Cre recombinase transgenic mouse. Genotypes were confirmed by sequencing and then PCR using the following primers: Forward: 5′-GGC GTT TAA AGA CGG ACA TAT AAC A-3′, Reverse: 5′-CCT CAA GGT CCA ATG CTC ATA C-3′. Biotinylation assay The anterior half of embryos collected at 17.5-days development (E17.5) from matings of ephrin-B2 lacZ/+ males and ephrin-B2 6YFΔV/+ females were dissociated with trypsin, and the resulting cell suspension was plated and allowed to grow in vitro for 24 hours. Cells were then exposed to sulfo-NHS-SS-biotin (Pierce no. 89881) to covalently link biotin to cell surface-exposed proteins, washed in growth media, and then total cell protein lysates were prepared in lysis buffer (1% Triton, 100mM NaCl, 50mM NaF, 50mM Tris–HCl pH 7.5) containing Complete (Roche) protease inhibitor cocktail. Streptavidin coated beads (Pierce) were used to pull down all biotinylated cell surface proteins, which were resolved on 6% Tris-glycine gels, transferred to PVDF (Millipore) membranes, and then immunoblotted with amino-terminal specific anti-ephrin-B2 (Neuromics) and anti-β-actin (Sigma) antibodies followed by secondary antibodies conjugated to horseradish peroxidase (Jackson). Histology and X-gal staining Embryos and postnatal pups were anesthetized, decapitated, washed in phosphate buffer, embedded in OCT and frozen in a slurry of dry ice and ethanol. Blocks were stored at −80 °C until cryosectioned at 14 μm onto Superfrost Plus (Fisher) slides. Sections were fixed in lacZ fixation solution (0.2% gluteraldehyde, 5 mM EGTA pH 7.3, 2 mM MgCl 2 in 0.1 M phosphate buffer) for 10 min followed by three 5 min washes in lacZ wash buffer (8 mM MgCl 2 , 0.08% Nonidet-P40 in 0.1 phosphate buffer). Sections were then stained in X-gal stain (2 ml of 25 mg ml −1 X-gal, 0.106 g potassium ferrocyanide, 0.082 g potassium ferricyanide in 50 ml wash buffer) overnight at 37°C. The next day, slides were washed twice for 5 min in lacZ wash buffer and fixed in 4% formalin for 5 min. After one wash for 5 min with PBS and then water, slides were immersed in Nuclear Fast Red for 45 s to label cell bodies. Slides were then washed for 10 min followed by ethanol dehydration, xylene clearing and slide cover mounting. Axon tracing and analysis Mice were anesthetized by hypothermia and DiI (Molecular Probes) solution (DiI crystals dissolved 5% in dimethylformamide) was injected into the dorsal or ventral peripheral retina at P6 as described previously [4] , [15] , [28] . On P8, pups were sacrificed, brains isolated, cortex removed, and contralateral SC whole mounts were analysed blind to genotype. Retinas from pups with DiI-labelled TZs in the SC were flatmounted to assess the injection site. Injection site was evaluated for position in relation to the four major eye muscles and containment of the DiI to the focal dorsal or ventral region desired. Flatmounted retinas and whole mount SC (boundaries determined by characteristic shape and location) were visualized using epifluorescence microscopy, CCD camera, and MetaVue software. DiI labelling of the optic tract path to the SC was observed at X2 and then the SC was visualized at X4 to evaluate the TZ(s) labelled. All results were analysed using the FET comparing the mutant to the wild-type group. Data was reported as distinct levels of significance (* P ≤0.05; ** P ≤0.01, and *** P ≤0.001). How to cite this article: Thakar, S. et al . Critical roles for EphB and ephrin-B bidirectional signalling in retinocollicular mapping. Nat. Commun. 2:431 doi: 10.1038/ncomms1445 (2011).